Epigenetic silencing ofOct4by a complex containing SUV39H1 andOct4pseudogene lncRNA Pseudogene-derived, long non-coding RNAs (lncRNAs) act as epigenetic regulators of gene expression. Here we present a panel of new mouse Oct4 pseudogenes and demonstrate that the X-linked Oct4 pseudogene Oct4P4 critically impacts mouse embryonic stem cells (mESCs) self-renewal. Sense Oct4P4 transcription produces a spliced, nuclear-restricted lncRNA that is efficiently upregulated during mESC differentiation. Oct4P4 lncRNA forms a complex with the SUV39H1 HMTase to direct the imposition of H3K9me3 and HP1α to the promoter of the ancestral Oct4 gene, located on chromosome 17, leading to gene silencing and reduced mESC self-renewal. Targeting Oct4P4 expression in primary mouse embryonic fibroblasts causes the re-acquisition of self-renewing features of mESC. We demonstrate that Oct4P4 lncRNA plays an important role in inducing and maintaining silencing of the ancestral Oct4 gene in differentiating mESCs. Our data introduces a sense pseudogene–lncRNA-based mechanism of epigenetic gene regulation that controls the cross-talk between pseudogenes and their ancestral genes. Oct4 is a member of the POU family of transcription factors that controls early embryonic differentiation and is essential to maintain mESC pluripotency and self-renewal [1] , [2] , [3] , [4] , [5] , [6] . Oct4 is expressed in germ cells, the inner cell mass of pre-implantation embryos, embryonic stem cells (ESC) but also in different types of human cancer [7] , [8] , [9] , [10] . Oct4 is essential to establish the core transcriptional network maintaining pluripotency and self-renewal in mESCs [1] , [2] , [3] , [4] . Importantly, ectopic expression of the key mESC self-renewal transcription factors Oct4 , Sox2 , Klf4 and c-Myc induces pluripotency in differentiated cells, resulting in induced pluripotent stem (iPS) cells [11] . Out of this basic set of transcription factors, Oct4 is the only indispensible factor for iPS cell generation [11] , [12] . This highlights a central role of Oct4 for ESC pluripotency and self-renewal. Given the key role of Oct4 in mESC self-renewal, discovering pathways that control Oct4 expression has primary importance. Induction of ESC differentiation leads to rapid transcriptional and epigenetic silencing of Oct4 (refs 13 , 14 , 15 , 16 , 17 , 18 ). Other pathways that regulate Oct4 expression involve post-translational modifications or miRNAs [19] , [20] , [21] , [22] , [23] , [24] , [25] . A growing body of evidence indicates an important role of pseudogene-derived RNAs in regulating the expression of their ancestral gene, either by modulating chromatin structure via anti-sense transcription, short interfering RNA (siRNA) formation or sponging miRNAs from their ancestral genes by acting as competing endogenous RNAs (ceRNAs) [26] , [27] , [28] , [29] , [30] , [31] , [32] . Recent studies demonstrate the existence of various human OCT4 pseudogenes and anticipate a relevance for pseudogene-derived ncRNAs in the regulation of the ancestral OCT4 gene in ESCs but also cancer [33] , [34] , [35] , [36] , [37] , [38] , [39] , [40] , [41] , [42] , [43] , [44] . To this end, the human OCT4 pseudogene OCT4-pg4 was demonstrated to sponge OCT4 -specific miRNAs in hepatocellular carcinoma cells [45] ; human OCT4-pg5 anti-sense transcripts reduce OCT4 promoter activity and mouse OCT4-pg1 impacts on mesenchymal stem cell differentiation via a still unknown mechanism [39] , [46] . However, the role of Oct4 pseuodogenes in controlling mESC pluripotency and self-renewal remains unknown. Here we identify a panel of novel, processed murine Oct4 pseudogenes and report on a trans -epigenetic cross-talk between an X-linked Oct4 pseudogene and the ancestral Oct4 gene, located on chromosome 17. We found that a long, non-coding RNA transcribed in sense orientation from Oct4 pseudogene 4 ( Oct4P4 ) recruits the H3K9-specific HMTase SUV39H1 to induce epigenetic repression of the promoter of the ancestral Oct4 gene in trans . This mechanism reduces the expression of key self-renewal transcription factors and promotes mESC differentiation. Importantly, functional disruption of the Oct4P4 –SUV39H1 silencing complex leads to a re-acquisition of self-renewal features, such as Oct4 expression and the re-activation of telomerase-dependent telomere maintenance mechanisms. This indicates that Oct4P4 is essential to prevent the re-activation of self-renewal circuits in differentiated cells. Oct4 pseudogenes expression during mESC differentiation Recent studies report the existence of eight OCT4 pseudogenes in the human and one Oct4 pseudogene ( Oct4-pg1 , here called ‘ Oct4P1 ’) in the mouse genome [36] , [38] , [39] , [40] . Performing genome blast analyses using the mouse Oct4 transcript 1 ( Pou5f1 ) complementary DNA (cDNA) as reference sequence, we identified four additional candidate pseudogenes ( Oct4P2, Oct4P3, Oct4P4 and Oct4P5 ) that show high homology to portions of the open reading frame and untranslated regions (UTRs) of the ancestral Oct4 transcript 1 ( Pou5f1 ) ( Fig. 1a ; Supplementary Fig. 1a ). Using primers specific for each Oct4 pseudogene, we were able to PCR amplify all candidate pseudogenes from random or oligo-dT primed cDNA prepared from mESC total RNA ( Fig. 1b ). No PCR product was obtained when cDNA synthesis was carried out in the absence of primers or reverse transcriptase, thus excluding RNA self-priming or contamination of PCR reactions with genomic DNA. The identity of all Oct4 pseudogene-derived RNAs was sequence validated ( Supplementary Fig. 1b ). We conclude that Oct4P2, Oct4P3, Oct4P4 and Oct4P5 represent novel, processed Oct4 pseudogenes that are expressed in mESCs. Interestingly, Oct4P4 shows homology to the entire mature Oct4 mRNA but has acquired a 334 bp insertion that shows high homology to the LTR element of the ERVL-MaLRs retrotransposon family ( Fig. 1a ). Remarkably, this insert is subjected to RNA splicing ( Supplementary Fig. 1c ). To test whether Oct4 pseudogenes are subjected to transcriptional regulation, we prepared total RNA from self-renewing mESC (EB T0) and mESCs that were subjected to embryoid body (EB) in vitro differentiation for 3 (EB D3), 5 (EB D5) or 7 (EB D7) days (see Supplementary information ). As expected, the ancestral Oct4 gene is subjected to efficient transcriptional repression during 7 days of EB differentiation ( Fig. 1c ). We found that EB differentiation is paralleled by a significant reduction of Oct4P1 and activation of Oct4P2 and Oct4P4 expression. EB differentiation does not significantly impact on Oct4P3 and Oct4P5 expression ( Fig. 1c ). Remarkably, Oct4P4 long non-coding RNA (lncRNA) levels are 150–300-fold higher in primary mouse embryonic fibroblasts (pMEFs) or immortalized mouse embryonic fibroblast compared with undifferentiated mESCs ( Fig. 1c ). Considering the lower RNA content of mESC compared with pMEFs [47] , we found that Oct4P4 lncRNA levels are more than 600-fold higher in pMEFs compared with mESCs ( Supplementary Fig. 1e ). Information on subcellular localization of lncRNAs can provide important information about a possible function as nuclear-restricted epigenetic regulator or cytoplasmatic ceRNA [27] , [48] . Pseudogene-specific quantitative reverse transcription–PCR (RT–PCR) using total RNA from nuclear and cytoplasmatic fractions of undifferentiated mESCs revealed that Oct4P2 and Oct4P4 are predominantly located in the nucleus ( Fig. 1d ). Oct4P1 , gapdh and the ancestral Oct4 mRNA show enrichment in the cytoplasm; Oct4P3 and Oct4P5 did not show specific enrichment in nucleus or cytoplasm of mESCs ( Fig. 1d ). Together, these data indicate that a subset of RNAs derived from Oct4 pseudogenes show controlled intracellular localization and tight transcriptional regulation, anticipating a potential role in the control of mESC self-renewal. Unique properties of the Oct4P4 lncRNA such as extended homology to the ancestral Oct4 gene, nuclear localization, splicing, efficient upregulation during mESC differentiation and the virtual absence of relevant ORFs ( Supplementary Fig. 1d ) prompted us to investigate a possible role of Oct4P4 in the control of mESC differentiation and self-renewal. 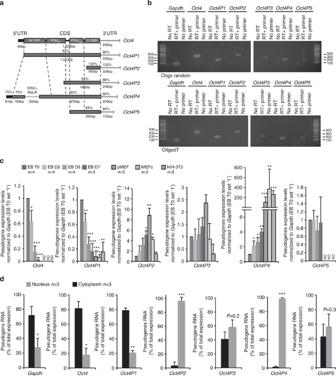Figure 1: Characterization of murineOct4pseudogenes. (a) Schematic representation ofOct4andOct4pseudogenes transcripts. Pseudogenes length and percentage of sequence homology to Oct4 are indicated. Regions with high homology to theOct45′UTR or 3′UTR are indicated by black boxes or grey lines, respectively. ERVL-MaLRs, spliced region ofOct4P4with homology to the LTR of ERVL-MaLRs retrotransposons. OCT4 protein domains are indicated: N-terminal trans-activating domain (N-TAD), POU-specific DNA-binding domain (POUs), DNA-binding homeodomain (POUHD), C-terminal trans-activating domain (C-TAD). (b) Verification ofOct4pseudogene expression in mouse embryonic stem cells (mESCs) by semi-quantitative PCR using random primed (top panel) or oligo-dT primed (bottom panel) cDNA. RT+primer, standard cDNA synthesis; no primer, cDNA synthesis without primers; no RT, cDNA synthesis without reverse transcriptase. PCR products are visualized on a 1.2% agarose gel. (c)Oct4lncRNA pseudogenes expression in self-renewing mESCs (EB T0) and embryoid body (EB) aggregates at day 3 (EB D3), day 5 (EB D5) and day 7 (EB D7); pMEFs; immortalized pMEFs and NIH-3T3 fibroblasts.Oct4pseudogenes expression was normalized togapdh. ND, not detectable. (d) Subcellular localization ofOct4pseudogene lncRNA in self-renewing mESCs. Expression values are shown as percentage of total RNA expression.n, number of independent experiments; error bars indicate s.d.; a Student’s t-test was used to calculate statistical significance values: *P<0.05; **P<0.01; ***P<0.001. Figure 1: Characterization of murine Oct4 pseudogenes. ( a ) Schematic representation of Oct4 and Oct4 pseudogenes transcripts. Pseudogenes length and percentage of sequence homology to Oct4 are indicated. Regions with high homology to the Oct4 5′UTR or 3′UTR are indicated by black boxes or grey lines, respectively. ERVL-MaLRs, spliced region of Oct4P4 with homology to the LTR of ERVL-MaLRs retrotransposons. OCT4 protein domains are indicated: N-terminal trans-activating domain (N-TAD), POU-specific DNA-binding domain (POU s ), DNA-binding homeodomain (POU HD ), C-terminal trans-activating domain (C-TAD). ( b ) Verification of Oct4 pseudogene expression in mouse embryonic stem cells (mESCs) by semi-quantitative PCR using random primed (top panel) or oligo-dT primed (bottom panel) cDNA. RT+primer, standard cDNA synthesis; no primer, cDNA synthesis without primers; no RT, cDNA synthesis without reverse transcriptase. PCR products are visualized on a 1.2% agarose gel. ( c ) Oct4 lncRNA pseudogenes expression in self-renewing mESCs (EB T0) and embryoid body (EB) aggregates at day 3 (EB D3), day 5 (EB D5) and day 7 (EB D7); pMEFs; immortalized pMEFs and NIH-3T3 fibroblasts. Oct4 pseudogenes expression was normalized to gapdh . ND, not detectable. ( d ) Subcellular localization of Oct4 pseudogene lncRNA in self-renewing mESCs. Expression values are shown as percentage of total RNA expression. n , number of independent experiments; error bars indicate s.d. ; a Student’s t-test was used to calculate statistical significance values: * P <0.05; ** P <0.01; *** P <0.001. Full size image Oct4P4 lncRNA represses the expression of ancestral Oct4 Next, we were interested in testing whether the existence of Oct4P4 sense and anti-sense transcripts could provide a possible inroad in understanding the role of Oct4P4 in mESC. Performing sense/anti-sense-specific RT–PCR, we were not able to detect anti-sense transcripts originating from the Oct4 and Oct4P4 genes. We therefore concluded that a putative function of Oct4P4 in mESCs must arise from Oct4P4 sense transcripts ( Supplementary Fig. 2a ). Investigating a possible role for Oct4P4 in mESC biology, we stably overexpressed sense Oct4P4 lncRNA in self-renewing mESCs. We found that stable overexpression of Oct4P4 resulted in a 23% reduction of alkaline phosphatase activity, a classic marker of mESC self-renewal potential ( Fig. 2a,b ). Remarkably, Oct4P4 overexpression reduced AP activity to a similar extent like RNA interference (RNAi)-mediated depletion of endogenous Oct4 ( Supplementary Fig. 2b,c ). Importantly, Oct4P4 overexpression caused a 50% reduction of OCT4 protein levels ( Fig. 2c ). Reduced alkaline phosphatase activity and OCT4 protein levels were found to be paralleled by significantly reduced mRNA expression of key pluripotency transcription factors such as Oct4 , Sox2 , Klf4 and Gdf3 and increased expression of early mESC differentiation markers such as Fgf5 , Brachyury , Nestin and Otx2 ( Fig. 2d ). Together, this indicates that ectopic expression of Oct4P4 impairs mESC self-renewal by interfering with transcriptional regulatory circuits that control pluripotency. 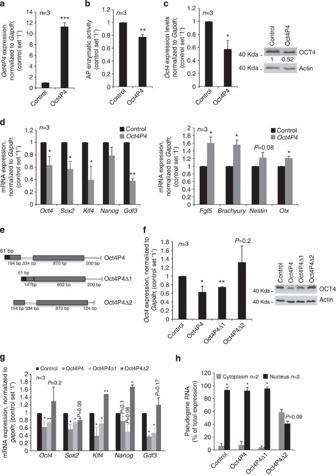Figure 2:Oct4P4impairs mESC self-renewal potential. (a) Quantitative real-time PCR determiningOct4P4lncRNA expression levels in mESCs stably overexpressingOct4P4.Oct4P4expression was normalized togapdh. (b) Spectrophotometric measurement of alkaline phosphatase (AP) activity in mESC stably overexpressingOct4P4. (c) EctopicOct4P4expression in self-renewing mESC reduces the expression ofOct4as determined by quantitative real-time PCR (left panel) or OCT4 western blotting (right panel). Expression values were normalized againstgapdh; ACTIN was used as a loading control in western blotting experiments. Numbers represent OCT4/ACTIN ratios (d) Quantitative real-time PCR analysis of self-renewal marker genes (left panel) or markers of early mESC differentiation (right panel) in mESCs stably overexpressingOct4P4. Expression levels were normalized againstGapdh. (e) Schematic representation of full-length andOct4P4deletion constructs. Oct4P4Δ1 lacks intronic ERVL-MaLR homology region and flanking sequences. Oct4P4Δ2 carries a 60 nt and 76 nt deletion at the 5′ and 3′ end of full-lengthOct4P4, respectively. (f) Quantitative real-time PCR analysis using mESCs stably overexpressingOct4P4,Oct4P4Δ1andOct4P4Δ2. Expression values were normalized againstgapdh(left panel). OCT4 western blotting analysis in mESCs stably overexpressingOct4P4, Oct4P4Δ1orOct4P4Δ2. ACTIN was used as a loading control (right panel).Oct4P4Δ2does not alter Oct4 expression. (g) Expression of pluripotency marker genes in mESCs ectopically expressingOct4P4,Oct4P4Δ1orOct4P4Δ2, as determined by quantitative real-time PCR analysis. Expression values were normalized againstgapdh. (h) Subcellular localization ofOct4P4,Oct4P4Δ1andOct4P4Δ2in mESCs stably expressing the indicated construct, as determined by real-time PCR. Expression values are shown as percentage of total expression.n, number of independent experiments carried out; error bars indicate s.d.; ND; not detected; a Student’st-test was used to calculate statistical significance values: *P<0.05; **P<0.01; ***P<0.001. Figure 2: Oct4P4 impairs mESC self-renewal potential. ( a ) Quantitative real-time PCR determining Oct4P4 lncRNA expression levels in mESCs stably overexpressing Oct4P4 . Oct4P4 expression was normalized to gapdh . ( b ) Spectrophotometric measurement of alkaline phosphatase (AP) activity in mESC stably overexpressing Oct4P4 . ( c ) Ectopic Oct4P4 expression in self-renewing mESC reduces the expression of Oct4 as determined by quantitative real-time PCR (left panel) or OCT4 western blotting (right panel). Expression values were normalized against gapdh ; ACTIN was used as a loading control in western blotting experiments. Numbers represent OCT4/ACTIN ratios ( d ) Quantitative real-time PCR analysis of self-renewal marker genes (left panel) or markers of early mESC differentiation (right panel) in mESCs stably overexpressing Oct4P4 . Expression levels were normalized against Gapdh . ( e ) Schematic representation of full-length and Oct4P4 deletion constructs. Oct4P4Δ1 lacks intronic ERVL-MaLR homology region and flanking sequences. Oct4P4Δ2 carries a 60 nt and 76 nt deletion at the 5′ and 3′ end of full-length Oct4P4 , respectively. ( f ) Quantitative real-time PCR analysis using mESCs stably overexpressing Oct4P4 , Oct4P4Δ1 and Oct4P4Δ2 . Expression values were normalized against gapdh (left panel). OCT4 western blotting analysis in mESCs stably overexpressing Oct4P4, Oct4P4Δ1 or Oct4P4Δ2 . ACTIN was used as a loading control (right panel). Oct4P4Δ2 does not alter Oct4 expression. ( g ) Expression of pluripotency marker genes in mESCs ectopically expressing Oct4P4 , Oct4P4Δ1 or Oct4P4Δ2 , as determined by quantitative real-time PCR analysis. Expression values were normalized against gapdh . ( h ) Subcellular localization of Oct4P4 , Oct4P4Δ1 and Oct4P4Δ2 in mESCs stably expressing the indicated construct, as determined by real-time PCR. Expression values are shown as percentage of total expression. n , number of independent experiments carried out; error bars indicate s.d. ; ND; not detected; a Student’s t -test was used to calculate statistical significance values: * P <0.05; ** P <0.01; *** P <0.001. Full size image To identify functionally relevant lncRNA domains, we created a panel of Oct4P4 expression vectors lacking Oct4P4 sequence elements with lowest sequence homology to the ancestral Oct4 cDNA ( Fig. 2e ). We found that stable overexpression of Oct4P4Δ1 that lacks a 449 nucleotide region comprising the 334 bp ERVL-MaLRs retrotransposon homology sequence was still able to reduce Oct4 mRNA and protein levels, recapitulating the effect of full-length Oct4P4 ( Fig. 2f ). In contrast, overexpression of Oct4P4Δ2, lacking sequences with high homology to the Oct4 5′ and 3′ UTR regions were not able to reduce Oct4 expression in mESCs ( Fig. 2f ). Oct4P4Δ1 overexpression significantly reduces the expression of pluripotency transcription factors. In contrast, Oct4P4Δ2 overexpression does not impact on self-renewing transcriptional circuits in self-renewing mESCs ( Fig. 2g ). These data suggest that Oct4P4 5′ and 3′UTR portions are important to reduce Oct4 expression. We therefore created additional Oct4P4 deletion constructs centred on regions located at the 5′ and 3′ termini of Oct4P4 lncRNA. Deleting the Oct4P4 -5′UTR (Oct4P4Δ5′UTR) or Oct4P4 -3′UTR (Oct4P4Δ3′UTR) resulted a reduced efficiency of Oct4 repression when compared with overexpression of full-length Oct4P4 lncRNA ( Supplementary Fig. 3a,b ). Ectopic expression of the 5′UTR or 3′UTR homology elements of the Oct4P4 lncRNA (Oct4P4-5′UTR or Oct4P4-3′UTR, respectively) did not impact on the expression of the ancestral Oct4 gene ( Supplementary Fig. 3c,d ). Together these data indicate that the 5′UTR and 3′UTR homology region of Oct4P4 collaborate to repress the expression of the ancestral Oct4 gene. Subcellular fractionation experiments revealed that ectopic Oct4P4 Δ 1 RNA maintains nuclear localization ( Fig. 2h ). In contrast, deletion of both, 5′ and 3′ UTR homology regions resulted in a non-specific subcellular distribution of Oct4P4 Δ 2 RNA in mESCs ( Fig. 2h ). Finally, individually deleting the 5′UTR or 3′UTR homology regions of Oct4P4 caused a reduced enrichment of Oct4P4Δ5′UTR or Oct4P4Δ3′UTR RNAs in the nucleus ( Supplementary Fig. 3e ). This indicates that the 5′UTR or 3′UTR are important to mediate nuclear localization of Oct4P4 . Of note, overexpression of Oct4P4 did not cause a subcellular de-localization of ancestral Oct4 or gapdh mRNAs, excluding that Oct4P4 impairs mESC self-renewal by de-localizing the ancestral Oct4 mRNA ( Supplementary Fig. 3f ). We conclude that the Oct4P4 pseudogene gives rise to a sense lncRNA that employs nuclear-restricted molecular mechanisms to reduce the expression of pluripotency transcription factors, finally leading to impaired mESC self-renewal. Oct4P4 lncRNA orchestrates silencing of the Oct4 promoter Based on the fact that nuclear localization is essential for Oct4P4 lncRNA function, we speculated that Oct4P4 might directly interact with the promoter of the ancestral Oct4 gene. To test this hypothesis, we performed Oct4 promoter luciferase reporter experiments in NIH-3T3 cells that lack expression of endogenous Oct4 ( Fig. 1c , Fig. 3a ). Co-transfection of the reporter with a plasmid-encoding haemagglutanin (HA)-epitope-tagged murine OCT4 under the control of the CMV promoter was able to increase Oct4 promoter luciferase reporter activity ( Fig. 3b , left panel). Importantly, Oct4P4 overexpression significantly attenuated this effect without affecting expression levels of ectopically expressed OCT4 protein ( Fig. 3b , right panel). This suggests that Oct4P4 -derived lncRNAs specifically reduced the activity of the Oct4 promoter used in the reporter construct. To provide evidence for a cross-talk between Oct4P4 ncRNA and the promoter of the ancestral Oct4 gene in trans , we established an ‘Oct4P4-MS2 RNA stem loop’ tethering system in mESC [49] . We generated mESCs stably co-expressing a flag-tagged version of MS2 phage coat protein (MS2-flag), as well as Oct4P4 lncRNA fused to 24 repeats of the MS2 RNA stem loop (24 × MS2 stem loop), that binds with high affinity to MS2 phage coat protein ( Fig. 3c ; Supplementary Material and Methods ). This model system permits the use of anti-flag antibodies to detect Oct4P4-24 × MS2 stem loop RNA at gene loci by chromatin immunoprecipitation (ChIP) or to identify Oct4P4 interacting proteins by RNA immunoprecipitation (RIP) ( Fig. 3c ). mESCs exclusively overexpressing MS2-flag were used as a control cells. In line with previous data, overexpression of MS2 stem loop-tagged Oct4P4 ( Oct4P4-24 × MS2 stem loop) results in reduced OCT4 protein and mRNA expression ( Fig. 3d ). Importantly, we were able to efficiently amplify Oct4P4-24 × MS2 stem loop RNA by RT–PCR in anti-flag RIP experiments using mESCs stably co-expressing MS2-flag and Oct4P4-24 × MS2 stem loop constructs. This demonstrates that MS2-flag forms a complex with the Oct4P4-24 × MS2 stem loop RNA in vivo ( Fig. 3e ). To demonstrate that Oct4P4-24 × MS2 stem loop RNA localizes to the endogenous Oct4 promoter region in MS2-flag expressing mESCs, we performed ChIP experiments using a set of primer pairs that specifically amplify the promoter of the ancestral Oct4 gene ( Fig. 3a ; primer pairs A, B) [50] . Performing ChIP using anti-flag antibodies, we were able to demonstrate the presence of MS2-Flag at the conserved Oct4 promoter/enhancer region CR2 in MS2-flag/ Oct4P4-24 × MS2 stem loop RNA-expressing mESCs ( Fig. 3f ). Importantly, MS2-flag control mESCs that lack Oct4P4-24 × MS2 stem loop RNA expression did not show association of MS2-flag with the Oct4 promoter ( Fig. 3f ). Anti-flag ChIP did not immunoprecipitate the promoter region of the unrelated Dkk gene in control cells ( Fig. 3f , right panel). 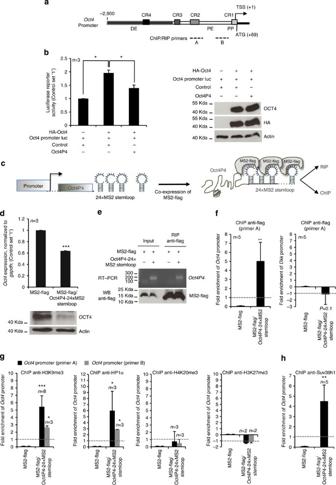Figure 3:Oct4P4mediates the imposition of H3K9me3 and HP1α at theOct4gene. (a) Schematic representation of the mouseOct4promoter region showing the location of the specific distal enhancer (DE), proximal enhancer (PE), proximal promoter (PP) sites and the conserved promoter/enhancer regions (CR1, CR2). The locations of PCR amplicons (A and B) used in ChIP experiments are indicated. (b) Luciferase reporter assay demonstrating thatOct4P4controlsOct4promoter activity. NIH-3T3 cells were co-transfected with indicated vectors. Luciferase activity was assayed 72 h after co-transfection (left panel); western blotting experiments using the indicated antibodies were performed in parallel (right panel). (c) Schematic representation of theOct4P4-24 × MS2stem loop construct used to generate mESCs stably expressing MS2-flag andOct4P4-24 × MS2stem loop RNA. (d)Oct4P4-24 × MS2stem loop RNA overexpression in mESC reduces the expression of ancestralOct4, as determined by quantitative RT–PCR; expression values were normalized againstGapdh(top panel); Result was validated by OCT4 western blotting, using ACTIN as a loading control (bottom panel). (e) RIP using mESCs overexpressing MS2-flag/Oct4P4-24 × MS2stem loop RNA or MS2-flag control cells. Agarose gel electrophoresis after semi-quantitative PCR demonstrates the presence ofOct4P4-24 × MS2stem loop RNA in anti-flag RIP experiments (top panel). Immunoprecipitation of MS2-flag was validated by western blotting (bottom panel) (f) ChIP using specific anti-flag antibodies followed by quantitative RT–PCR using lysates from MS2-flag/Oct4P4-24 × MS2stem loop or MS2-flag control mESCs. MS2-flag is enriched at theOct4promoter inOct4P4-24 × MS2stem loop mESCs (left panel); no enrichment was detected at the unrelatedDkkpromoter (right panel). ChIP data were quantified versus input and unrelated HA-specific antibodies. (g) ChIP analysis ofOct4promoter region in mESCs stably overexpressingOct4P4using indicated antibodies. Quantitative RT–PCR was performed to measure promoter enrichment.Oct4P4overexpression drives H3K9me3 and HP1α enrichment at Oct4 promoter region. (h) ChIP analysis ofOct4promoter region in MS2-flag/Oct4P4-24 × MS2stem loop and control MS2-flag mESCs using SUV39H1-specific antibodies.Oct4P4-24 × MS2stem loop results in an enrichment of SUV39H1 at theOct4promoter.n, number of independent experiments carried out; WB, western blotting; error bars indicate s.d.; a Student’st-test was used to calculate statistical significance values: *P<0.05; **P<0.01; ***P<0.001. Figure 3: Oct4P4 mediates the imposition of H3K9me3 and HP1α at the Oct4 gene. ( a ) Schematic representation of the mouse Oct4 promoter region showing the location of the specific distal enhancer (DE), proximal enhancer (PE), proximal promoter (PP) sites and the conserved promoter/enhancer regions (CR1, CR2). The locations of PCR amplicons (A and B) used in ChIP experiments are indicated. ( b ) Luciferase reporter assay demonstrating that Oct4P4 controls Oct4 promoter activity. NIH-3T3 cells were co-transfected with indicated vectors. Luciferase activity was assayed 72 h after co-transfection (left panel); western blotting experiments using the indicated antibodies were performed in parallel (right panel). ( c ) Schematic representation of the Oct4P4-24 × MS2 stem loop construct used to generate mESCs stably expressing MS2-flag and Oct4P4-24 × MS2 stem loop RNA. ( d ) Oct4P4-24 × MS2 stem loop RNA overexpression in mESC reduces the expression of ancestral Oct4 , as determined by quantitative RT–PCR; expression values were normalized against Gapdh (top panel); Result was validated by OCT4 western blotting, using ACTIN as a loading control (bottom panel). ( e ) RIP using mESCs overexpressing MS2-flag/ Oct4P4-24 × MS2 stem loop RNA or MS2-flag control cells. Agarose gel electrophoresis after semi-quantitative PCR demonstrates the presence of Oct4P4-24 × MS2 stem loop RNA in anti-flag RIP experiments (top panel). Immunoprecipitation of MS2-flag was validated by western blotting (bottom panel) ( f ) ChIP using specific anti-flag antibodies followed by quantitative RT–PCR using lysates from MS2-flag/ Oct4P4-24 × MS2 stem loop or MS2-flag control mESCs. MS2-flag is enriched at the Oct4 promoter in Oct4P4-24 × MS2 stem loop mESCs (left panel); no enrichment was detected at the unrelated Dkk promoter (right panel). ChIP data were quantified versus input and unrelated HA-specific antibodies. ( g ) ChIP analysis of Oct4 promoter region in mESCs stably overexpressing Oct4P4 using indicated antibodies. Quantitative RT–PCR was performed to measure promoter enrichment. Oct4P4 overexpression drives H3K9me3 and HP1α enrichment at Oct4 promoter region. ( h ) ChIP analysis of Oct4 promoter region in MS2-flag/ Oct4P4-24 × MS2 stem loop and control MS2-flag mESCs using SUV39H1-specific antibodies. Oct4P4-24 × MS2 stem loop results in an enrichment of SUV39H1 at the Oct4 promoter. n , number of independent experiments carried out; WB, western blotting; error bars indicate s.d. ; a Student’s t -test was used to calculate statistical significance values: * P <0.05; ** P <0.01; *** P <0.001. Full size image Together, our data demonstrate that the Oct4P4 lncRNA is required to localize MS2-flag to the Oct4 promoter in MS2-flag/Oct4P4-24 × MS2 stem loop RNA-expressing mESCs. This data support a model where a sense-oriented Oct4P4 lncRNA can localize in trans to the promoter of the Oct4 gene. Nuclear, lncRNAs such as XIST , HOTAIR or pericentric satellite repeats plays a key role in recruiting epigenetic repressors such as the H3K9-specific SUV39H Histone HMTases or H3K27-specific HMTase containing Polycomb repressive complexes [51] , [52] , [53] . We consequently speculated that upregulation of Oct4P4 ncRNA expression during mESC differentiation ( Fig. 1c ) might direct epigenetic silencing complexes to the endogenous Oct4 promoter. Taking advantage of our Oct4P4 -MS2 RNA tethering mESC model system, we found that Oct4P4-24 × MS2 stem loop RNA overexpression in MS2-flag mESCs result in a fivefold increase of H3K9me3 at conserved Oct4 promoter/enhancer regions (CR1, CR2; detected by primer pairs A and B), as determined by ChIP ( Fig. 3a,g ). Consistent with the reported high binding affinity of HP1 to H3K9me3 (ref. 54 ), we found a sixfold increase of HP1α at the Oct4 promoter in our model mESC line ( Fig. 3g ). Of note, Oct4P4-24 × MS2 stem loop RNA overexpression in MS2-flag mESCs does not impact on the abundance of H4K20me3 or H3K27me3 at the Oct4 promoter ( Fig. 3g ). In line with increased H3K9me3 levels, we found a fourfold increase of the H3K9-specific SUV39H1 HMTase at the Oct4 promoter of MS2-flag/ Oct4P4-MS2-24 × MS2 stem loop mESCs ( Fig. 3h ). To individuate Oct4P4 lncRNA regions that are important for SUV39H1 interaction and SUV39H1 deposition on the Oct4 promoter, we performed anti-SUV39H1 ChIP and RIP experiments using mESCs stably overexpressing full-length Oct4P4, Oct4P4Δ5′UTR , Oct4P4Δ3′UTR or Oct4P4Δ2 lncRNAs. Importantly, we found that SUV39H1 deposition on the Oct4 promoter was reduced in Oct4P4Δ5′UTR and Oct4P4Δ3′UTR cells when compared with full-length Oct4P4 overexpressing cells ( Supplementary Fig. 4a ). Deletion of the Oct4 5′ and 3′ UTR homology regions in Oct4P4 reduced efficiency of Oct4P4 lncRNA mediated repression of Oct4 ( Fig. 2f ). In line with this, mESCs overexpressing Oct4P4 lncRNAs lacking the 5′UTR ( Oct4P4Δ5′UTR ) or 3′UTR ( Oct4P4Δ3′UTR ) homology show reduced SUV39H1 abundance at the Oct4 promoter when compared with cells overexpressing the full-length Oct4P4 lncRNA ( Supplementary Fig. 4a ). Finally, overexpression of an Oct4P4 version lacking both the 3′ and 5′ UTR homology region (Oct4P4Δ2) did not result in the accumulation of SUV39H1 at the Oct4 promoter. This indicates that the 5′ and 3′UTR homology regions are important to localize SUV39H1 to the Oct4 promoter. Accordingly, Oct4P4Δ2 was no longer able to physically interact with SUV39H1 ( Supplementary Fig. 4b ), further underlying the importance of 5′ UTR and 3′UTR homology regions for Oct4P4 function. Altogether, our data show that the Oct4P4 lncRNA, expressed in sense orientation from X-linked Oct4P4 locus, mediates the enrichment of H3K9me3, HP1α and SUV39H1 at the Oct4 promoter, located on chromosome 17. This trans- acting silencing mechanism leads to reduced Oct4 expression that finally results in impaired self-renewal potential of mESCs ( Fig. 3d,g,h ). An Oct4P4 –SUV39H1 complex targets the Oct4 promoter We showed that Oct4P4 lncRNA overexpression leads to chromatin compaction at the promoter of the ancestral Oct4 gene. We next wished to test whether (i) Oct4P4 physically interacts with SUV39H1 and (ii) both players are required to induce epigenetic gene silencing at the promoter of the ancestral Oct4 gene. Using MS2-flag/ Oct4P4-24 × MS2 stem loop model mESC, we found that anti-SUV39H1-specific antibodies were able to immunoprecipitate MS2-flag but also Oct4P4-24 × MS2 stem loop lncRNA ( Fig. 4a ; Supplementary Fig. 5a ). Importantly, also endogenous Oct4P4 lncRNA was detectable by RT–PCR in anti-SUV39H1 RIP experiments using pMEFs, that are characterized by high Oct4P4 lncRNA expression levels ( Figs 1c and 4b ). Of note, Oct4P4 lncRNA abundance was found to be strongly reduced in anti-SUV39H1 RNA immunoprecipitates after RNAi-mediated reduction of endogenous Oct4P4 , thus confirming the specificity of our experiments ( Fig. 4b ). 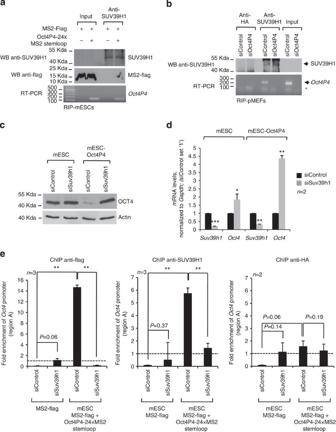Figure 4:Oct4P4interacts with SUV39H1 to silence ancestralOct4intrans. (a) Anti-SUV39H1 RIP using MS2-flag/Oct4P4-24 × MS2stem loop mESCs or MS2-flag mESCs cells. Efficiency of anti-SUV39H1 immunoprecipitation was validated by western blotting (top panel). SUV39H1 is not detectable in inputs due to reduced antibody efficiency in western blotting compared with immunoprecipitation (Supplementary Fig. 5a). MS2-flag co-immunoprecipitates with SUV39H1 only in the presence ofOct4P4-24 × MS2stem loop RNA, as determined by western blotting (middle panel). Semi-quantitative RT–PCR followed by agarose gel electrophoresis verified the presence ofOct4P4-24 × MS2-stem loop RNA in anti-SUV39H1 RIP (bottom panel). (b) Anti-SUV39H1 RIP immunoprecipitation of endogenousOct4P4RNA from lysates obtained from pMEFs transfected with control or Suv39h1-specific siRNAs. Efficiency of SUV39H1 immunoprecipitation was validated by western blotting (top panel).Oct4P4RNA is undetectable in RIP experiments using lysates fromSuv39h1depleted cells, demonstrating the specificity of the anti-SUV39H1 antibody (bottom panel). A human influenza haemagglutinin (HA) antibody was used as a control in RIP experiments. (c,d)Oct4expression levels in wild-type (wt) mESCs and mESCs stably overexpressingOct4P4after transient transfected with the indicated siRNA oligos.Suv39h1 knockdown increasesOct4expression on the protein (c) and mRNA level (d) as determined by western blotting (c) and quantitative real-time PCR (d). ACTIN was used as a loading control in western blotting;Oct4mRNA levels were normalized togapdh. (e)Oct4promoter ChIP using MS2-flag control and MS2-flag/Oct4P4-24 × MS2stem loop mESCs underSuv39h1knock-down conditions. Quantitative real-time PCR on anti-flag immunoprecipitates demonstrates that aOct4P4-24 × MS2stem loop/MS2-flag RNA–protein complex associates with the endogenousOct4promoter only in the presence ofSuv39h1(left panel).Suv39h1knockdown significantly reduces SUV39H1 abundance at the Oct4 promoter, demonstrating specificity of the anti-SUV39H1 antibody (middle panel). An HA antibody was used as a control (right panel).Dkkpromoter was used as a negative control.n, number of independent experiments carried out; WB, western blotting; error bars indicate s.d.; a Student’st-test was used to calculate statistical significance values: *P<0.05; **P<0.01; ***P<0.001. Figure 4: Oct4P4 interacts with SUV39H1 to silence ancestral Oct4 in trans . ( a ) Anti-SUV39H1 RIP using MS2-flag /Oct4P4-24 × MS2 stem loop mESCs or MS2-flag mESCs cells. Efficiency of anti-SUV39H1 immunoprecipitation was validated by western blotting (top panel). SUV39H1 is not detectable in inputs due to reduced antibody efficiency in western blotting compared with immunoprecipitation ( Supplementary Fig. 5a ). MS2-flag co-immunoprecipitates with SUV39H1 only in the presence of Oct4P4-24 × MS2 stem loop RNA, as determined by western blotting (middle panel). Semi-quantitative RT–PCR followed by agarose gel electrophoresis verified the presence of Oct4P4-24 × MS2- stem loop RNA in anti-SUV39H1 RIP (bottom panel). ( b ) Anti-SUV39H1 RIP immunoprecipitation of endogenous Oct4P4 RNA from lysates obtained from pMEFs transfected with control or Suv39h1-specific siRNAs. Efficiency of SUV39H1 immunoprecipitation was validated by western blotting (top panel). Oct4P4 RNA is undetectable in RIP experiments using lysates from Suv39h1 depleted cells, demonstrating the specificity of the anti-SUV39H1 antibody (bottom panel). A human influenza haemagglutinin (HA) antibody was used as a control in RIP experiments. ( c , d ) Oct4 expression levels in wild-type (wt) mESCs and mESCs stably overexpressing Oct4P4 after transient transfected with the indicated siRNA oligos. Suv39h 1 knockdown increases Oct4 expression on the protein ( c ) and mRNA level ( d ) as determined by western blotting ( c ) and quantitative real-time PCR ( d ). ACTIN was used as a loading control in western blotting; Oct4 mRNA levels were normalized to gapdh . ( e ) Oct4 promoter ChIP using MS2-flag control and MS2-flag/ Oct4P4-24 × MS2 stem loop mESCs under Suv39h1 knock-down conditions. Quantitative real-time PCR on anti-flag immunoprecipitates demonstrates that a Oct4P4-24 × MS2 stem loop/MS2-flag RNA–protein complex associates with the endogenous Oct4 promoter only in the presence of Suv39h1 (left panel). Suv39h1 knockdown significantly reduces SUV39H1 abundance at the Oct4 promoter, demonstrating specificity of the anti-SUV39H1 antibody (middle panel). An HA antibody was used as a control (right panel). Dkk promoter was used as a negative control. n , number of independent experiments carried out; WB, western blotting; error bars indicate s.d. ; a Student’s t -test was used to calculate statistical significance values: * P <0.05; ** P <0.01; *** P <0.001. Full size image Next, we wished to validate that SUV39H1 is required to reduce Oct4 expression by mediating the enrichment of H3K9me3 and its high-affinity binding partner HP1α at the Oct4 promoter. RNAi-mediated knockdown of SUV39H1 resulted in significantly increased Oct4 mRNA and OCT4 protein levels in wild-type mESCs and Oct4P4 lncRNA-overexpressing mESCs. This provided first evidence that the SUV39H1 HMTase controls Oct4 expression in mESCs ( Fig. 4c,d ). To understand the relevance of SUV39H1 for the establishment of a repressive chromatin structure at the endogenous Oct4 promoter, we performed anti-flag and anti-SUV39H1 ChIP experiments in MS2-flag/ Oct4P4-24 × MS2 stem loop mESCs. As expected, SUV39H1 RNAi resulted in reduced abundance of SUV39H1 and H3K9me3 at the Oct4 promoter in MS2-flag/ Oct4P4-24 × MS2 stem loop mESCs ( Fig. 4e , Supplementary Fig. 5b ). Importantly, this effect was paralleled by reduced MS2-flag levels at the Oct4 promoter, indicative for reduced abundance of Oct4P4-24 × MS2 stem loop RNA at the ancestral Oct4 promoter. Together, this indicates that both SUV39H1 and Oct4P4 lncRNA are required to mediate localization of the silencing complex to the endogenous Oct4 promoter. Oct4P4 blocks aberrant acquisition of self-renewal features High Oct4P4 lncRNA expression levels in pMEFs ( Fig. 1c ) suggest that the Oct4P4 –SUV39H1 lncRNA–protein complex has an important role in silencing the endogenous Oct4 promoter in differentiated cells. In line with this hypothesis, we found that siRNA-mediated knockdown of Oct4P4 lncRNA in pMEFs results in a fourfold or twofold reduction of SUV39H1 or H3K9me3 at the Oct4 promoter, respectively ( Fig. 5a,b ). Importantly, reduced chromatin compaction at the Oct4 promoter was paralleled by a significant increase in Oct4 mRNA expression ( Fig. 5c ). This data was confirmed in experiments using an independent Oct4P4 lncRNA-specific siRNA oligonucleotide ( Supplementary Fig. 6a,b ). This indicates that the Oct4P4 –SUV39H1 complex plays an important role in maintaining silencing of the Oct4 promoter in pMEFs. Interestingly, we found that Oct4P4 is efficiently repressed during the conversion of pMEFs to iPS ( Fig. 5d ). This suggests that Oct4P4 might represent a barrier to the de-differentiation of pMEFs. To further test this idea, we performed Oct4P4 loss-of-function experiments in pMEFs. Oct4P4 knockdown caused a change of the characteristic flat and single-cell morphology of pMEFs to round-shaped cells but also the formation of multi-cellular spheres that grow in suspension or attached on top of pMEFs ( Fig. 5e ). The formation of spheres or round-shaped cells was inhibited when pMEFs were co-transfected with a mix of siOct4P4 and siOct4 oligonucleotides, indicating that changes in cell morphology are Oct4 dependent ( Fig. 5e,f ). Importantly, siOct4P4-induced changes in cell morphology were paralleled by a significantly increased expression of mESC pluripotency transcription factors Oct4 (threefold), Sox2 (threefold), Nanog (threefold) and Klf4 (twofold) ( Fig. 5f ). This data was confirmed in experiments using an independent Oct4P4 -specific siRNA oligonucleotide ( Supplementary Fig. 6c ). Remarkably, siOct4P4-dependent increase of pluripotency transcription factor expression was attenuated by contemporary knockdown of Oct4 ( Fig. 5f ). Together, this indicates that depletion of Oct4P4 from pMEFs results in a loss of heterochromatin at the Oct4 promoter, leading to the re-activation of endogenous Oct4 that promotes the expression of additional key transcription factors of mESC self-renewal. To find evidence that loss of Oct4P4 activates other biological pathways linked to mESC self-renewal programmes, we studied the impact of Oct4P4 on telomere maintenance in pMEFs. pMEFs are characterized by progressive telomere shortening due to lack of sufficient telomerase activity. In line with this, re-activation of telomerase activity is a key step for the acquisition of pluripotency during iPS reprogramming of pMEFs [55] . Importantly, we found that 2 consecutive cycles of RNAi-mediated depletion of Oct4P4 from pMEFs resulted in a 2.6-fold upregulation of the transcript for the catalytic subunit of telomerase, TERT. Importantly, Tert mRNA upregulation was paralleled by a concomitant increase in telomeric DNA repeat content, as determined by real-time PCR-based quantification of telomeric DNA repeats in experimental cells ( Fig. 5g,h ). This data was confirmed in experiments using independent Oct4P4 -specific siRNA oligonucleotides ( Supplementary Fig. 6c,d ). This indicates that Oct4P4 depletion re-activates telomerase expression to drive telomere elongation. Remarkably, these effects were attenuated when pMEFs where transfected with a mix of siRNAs that target Oct4P4 lncRNA and the ancestral Oct4 mRNA ( Fig. 5g,h ). 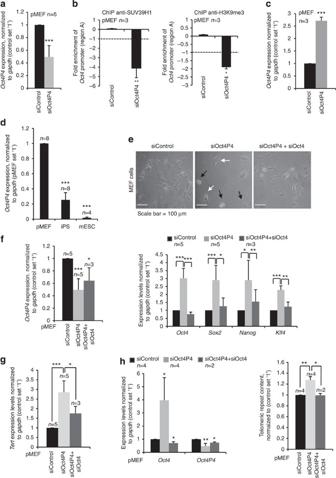Figure 5:Oct4P4prevents the activation of features of mESC self-renewal in pMEFs. (a) Quantitative real-time PCR determiningOct4P4expression levels in pMEFs transiently transfected with siRNA targetingOct4P4. Control cells were transfected with siRNA control oligos.Oct4P4expression was normalized togapdh. (b)Oct4promoter ChIP analysis using SUV39H1- or H3K9me3-specific antibodies in MEFs transiently transfected with indicated siRNAs.Oct4P4siRNA reduces H3K9me3 and SUV39H1 abundance, at theOct4promoter, as determined by quantitative real-time PCR (Oct4amplicon A). Dkk promoter was used as a negative control. (c) siRNA-mediated knockdown ofOct4P4in pMEFs increasesOct4expression in quantitative real-time PCR experiments. Expression values were normalized againstgapdh. (d)Oct4P4lncRNA expression in pMEFs and their derivative iPS cells. mESCs were included as control.Oct4P4expression levels were normalized againstgapdh. (e) Morphology of pMEFs transfected with the indicated siRNAs oligonucleotides. Black arrows indicate cells with altered cell morphology. White arrows indicate pMEFs. Scale bar, 100 μm (f) Quantitative real-time PCR analysis ofOct4P4lncRNA levels (left panel) and mESC self-renewal marker genes (right panel) in pMEFs transiently transfected with siRNA targetingOct4P4or with a combination of siOct4P4 and siOct4 oligonucleotides. Expression levels were normalized againstgapdh. Knockdown ofOct4P4causes an increased expression of self-renewal marker genes. Reduction ofOct4expression in the context ofOct4P4knockdown rescues self-renewal marker genes. (g)TertmRNA expression level in pMEFs transfected with indicated siRNA oligonucleotides, as determined by quantitative real-time PCR. siRNA-mediated knockdown ofOct4P4increasesTertexpression. Expression levels were normalized againstgapdh. (h) Measurement of telomere repeat content by quantitative real-time PCR. Total genomic DNA from pMEF transiently transfected with indicated siRNA oligonucleotides were analysed using telomere repeat-specific PCR primers (right panel). Alu-equivalent B1 repeats were used as a reference sequence. siRNA-mediated reduction ofOct4P4leads to increased telomere repeat content, indicative for increased telomere length. Knock-down efficiency was validated by quantitative RT–PCR (left panel).n, the number of independent experiments carried out; error bars indicate s.d.; a Student’st-test was used to calculate statistical significance values: *P<0.05; **P<0.01; ***P<0.001. Figure 5: Oct4P4 prevents the activation of features of mESC self-renewal in pMEFs. ( a ) Quantitative real-time PCR determining Oct4P4 expression levels in pMEFs transiently transfected with siRNA targeting Oct4P4 . Control cells were transfected with siRNA control oligos. Oct4P4 expression was normalized to gapdh . ( b ) Oct4 promoter ChIP analysis using SUV39H1- or H3K9me3-specific antibodies in MEFs transiently transfected with indicated siRNAs. Oct4P4 siRNA reduces H3K9me3 and SUV39H1 abundance, at the Oct4 promoter, as determined by quantitative real-time PCR ( Oct4 amplicon A). Dkk promoter was used as a negative control. ( c ) siRNA-mediated knockdown of Oct4P4 in pMEFs increases Oct4 expression in quantitative real-time PCR experiments. Expression values were normalized against gapdh . ( d ) Oct4P4 lncRNA expression in pMEFs and their derivative iPS cells. mESCs were included as control. Oct4P4 expression levels were normalized against gapdh . ( e ) Morphology of pMEFs transfected with the indicated siRNAs oligonucleotides. Black arrows indicate cells with altered cell morphology. White arrows indicate pMEFs. Scale bar, 100 μm ( f ) Quantitative real-time PCR analysis of Oct4P4 lncRNA levels (left panel) and mESC self-renewal marker genes (right panel) in pMEFs transiently transfected with siRNA targeting Oct4P4 or with a combination of siOct4P4 and siOct4 oligonucleotides. Expression levels were normalized against gapdh . Knockdown of Oct4P4 causes an increased expression of self-renewal marker genes. Reduction of Oct4 expression in the context of Oct4P4 knockdown rescues self-renewal marker genes. ( g ) Tert mRNA expression level in pMEFs transfected with indicated siRNA oligonucleotides, as determined by quantitative real-time PCR. siRNA-mediated knockdown of Oct4P4 increases Tert expression. Expression levels were normalized against gapdh . ( h ) Measurement of telomere repeat content by quantitative real-time PCR. Total genomic DNA from pMEF transiently transfected with indicated siRNA oligonucleotides were analysed using telomere repeat-specific PCR primers (right panel). Alu-equivalent B1 repeats were used as a reference sequence. siRNA-mediated reduction of Oct4P4 leads to increased telomere repeat content, indicative for increased telomere length. Knock-down efficiency was validated by quantitative RT–PCR (left panel). n , the number of independent experiments carried out; error bars indicate s.d. ; a Student’s t -test was used to calculate statistical significance values: * P <0.05; ** P <0.01; *** P <0.001. Full size image Together, our data demonstrate that depleting Oct4P4 from differentiated pMEFs results in the re-activation of basic features of mESC pluripotency, such as self-renewal transcription factor expression and activation of telomerase-dependent mechanisms of telomere maintenance. This further indicates that Oct4P4 has an important role in preventing the aberrant expression of self-renewal promoting transcription factors in differentiated cells. Pseudogene-derived transcripts have been reported to impact on the expression of ancestral protein-coding gene using molecular pathways based on RNA sequence homology. Pseudogenes derived transcripts were demonstrated to control ancestral gene by producing endogenous siRNAs, sponging miRNAs by acting as ceRNAs or altering the stability of the ancestral mRNA [28] , [29] , [30] , [31] , [32] , [56] . In addition, anti-sense pseudogene transcripts can impact on the promoter activity of ancestral genes [30] , [36] , [57] , [58] . In this study, we used mESCs to identify a set of novel transcripts derived from putative Oct4 pseudogenes ( Oct4P1, Oct4P2, Oct4P3 Oct4P4 and Oct4P5 ). Tight regulation of subcellular localization and expression during mESC differentiation anticipate a defined role for a subset of these transcripts in mESC biology. Here we focused our studies on a nuclear-restricted non-coding RNA (ncRNA) that is transcribed in sense orientation from the processed, X-linked Oct4P4 . Dramatic upregulation of sense Oct4P4 transcription during mESC differentiation gives rise to a long, non-coding RNA that forms a complex with the repressive H3K9-specific HMTase SUV39H1. This complex translocates to the promoter of the ancestral Oct4 protein-coding gene, located on chromosome 17, to impose H3K9 tri-methylation leading to a consecutive recruitment of HP1α and silencing of the ancestral Oct4 gene ( Fig. 6 ). This is in a remarkable contrast to the ceRNA function of the human cytoplasmatic lncRNA OCT4-pg4 in hepatocellular carcinoma [45] . Thus murine Oct4P4 and human OCT4-pg4 are not mechanistically conserved and act via completely different cellular pathways. A recent study reported that anti-sense transcripts originating from the human OCT4-pg5 can mediate silencing of the human OCT4 gene in cancer cells [46] . Importantly, we were not able to detect anti-sense transcripts originating from murine ancestral Oct4 or Oct4P4 genes ( Supplementary Fig. 2a ). We also did not find a significant homology between the Oct4P4 lncRNA and the Oct4 promoter ( Supplementary Fig. 7c ). Finally, O ct4P4 lncRNA did not impact on Oct4P4 promoter activity ( Supplementary Fig. 7a,b ). Thus, these findings do not support a model that involves the expression of an anti-sense Oct4P4 transcript or direct interaction of Oct4P4 lncRNA with the Oct4 promoter that is based on sequence homology. We rather propose that sense-oriented Oct4P4 lncRNAs represents the functionally relevant pseudogene-derived lncRNA that forms a complex with SUV39H1 and then translocates to the promoter of the ancestral Oct4 gene. In line with this, deleting Oct4P4 5′ or 3′ sequences that show high homology to the 5′UTR or 3′UTR regions, respectively, of ancestral Oct4 significantly reduce the ability of Oct4P4 lncRNA to deposit SUV39H1 at the Oct4 promoter, thus leading to reduced Oct4 silencing. This highlights a possible importance of 5′UTR and 3′UTR homology regions of pseudogene-derived sense transcripts for epigenetic gene regulation. 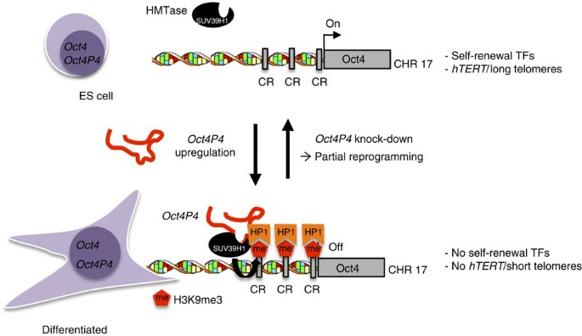Figure 6:A model forOct4P4lncRNA function. The nuclear, long non-codingOct4P4is upregulated during mESC differentiation and recruits the H3K9-specific HMTase SUV39H1 to impose H3K9me3 and HP1α at the promoter of ancestralOct4gene intrans, leading toOct4gene silencing. Depletion ofOct4P4lncRNA in differentiated pMEFs results in re-activation ofOct4expression and the acquisition of classic features of self-renewal such as increased expression of self-renewal transcription factors and activation of telomerase-dependent telomere maintenance mechanisms. This indicates thatOct4P4prevents the aberrant expression of self-renewal programmes in differentiated cells. Figure 6: A model for Oct4P4 lncRNA function. The nuclear, long non-coding Oct4P4 is upregulated during mESC differentiation and recruits the H3K9-specific HMTase SUV39H1 to impose H3K9me3 and HP1α at the promoter of ancestral Oct4 gene in trans , leading to Oct4 gene silencing. Depletion of Oct4P4 lncRNA in differentiated pMEFs results in re-activation of Oct4 expression and the acquisition of classic features of self-renewal such as increased expression of self-renewal transcription factors and activation of telomerase-dependent telomere maintenance mechanisms. This indicates that Oct4P4 prevents the aberrant expression of self-renewal programmes in differentiated cells. Full size image Remarkably, the human OCT4-pg3 (here OCT4P3 , NR_036440.1), OCT4-pg4 (here OCT4P4 , NR_034180.1) and OCT4-pg1 (here OCT4P1b NM_001159542.1) show homology to the entire OCT4 cDNA and share high structural and sequence homology to murine Oct4P4 . Similar to Oct4P4 in mESCs, we found that human OCT4P3 lncRNA is enriched in the nuclei of OVCAR-3 and SKOV-3 ovarian cancer cells ( Supplementary Fig. 8 ). This provides a first indication for a possible conservation of Oct4P4/OCT4P3 function. Interfering with the murine Oct4P4 –SUV39H1 silencing complex in differentiated cells leads to the re-activation of mESC self-renewal transcription factor expression and telomerase-dependent telomere maintenance mechanism ( Fig. 6 ). This represents a partial re-acqusition of mESC stem cell features in short term (6 days) Oct4P4 lncRNA knock-down experiments. It will be interesting to test whether loss of Oct4P4 function can increase the efficiency of iPS cell generation protocols. Together, our data indicates that Oct4P4 and SUV39H1 are important to prevent the aberrant activation of mESCs self-renewal pathways in differentiated cells. Future experiments will aim to better define structural Oct4P4 lncRNA motifs involved in SUV39H1 recruitment and elucidate pathways that direct Oct4P4 to the ancestral Oct4 gene. Several lncRNAs such as XIST or HOTAIR have been described to act as scaffold for the formation of chromatin-modifying complexes [51] , [52] . To our knowledge, the Oct4P4 lncRNA represents the first example for a crucial role of a vertebrate pseudogene-derived sense lncRNAs in directing chromatin-modifying activities to the promoter of its ancestral gene in trans . Given the vast repertoire of vertebrate pseudogenes, we anticipate the existence of a series of pseudogene-derived lncRNAs that use mechanisms analogous to Oct4P4 to control the expression of ancestral genes on the epigenetic level. Understanding pseudogene lncRNA-dependent mechanism of epigenetic gene regulation and a precise categorization of pseudogene-derived lncRNAs based on subcellular localization, gene expression regulation and deposition at gene promoters will provide important insights into the global role of pseudogene-derived lncRNAs in regulating higher order chromatin structures. Cell culture and generation of stable cell lines Feeder-independent mouse ESCs [59] were cultured on gelatin (0.2%) coated plates in mESC self-renewal medium (DMEM with 15% knockout serum replacement (Gibco), 1% nonessential amino acids (Gibco), 1 mM sodium pyruvate (Invitrogen), 1% L-glutamine (Invitrogen), 0.1 mM ß-mercaptoethanol, 1% penicillin/streptomycin (Invitrogen) and 1,000 U ml −1 mouse leukaemia inhibitory factor. pMEFs were generated from 13.5 d.p.c C57BL/6 mouse embryos. NIH-3T3 cells were obtained from ATCC. pMEFs and NIH-3T3 cells were maintained in culture in DMEM supplemented with 10% foetal bovine serum (Lonza) and 1% penicillin/streptomycin. iPS were generated and cultivated according to standard conditions [60] . OVCAR-3 cells (ATCC) were cultured in RPMI-1640 medium supplemented with 20% foetal bovine serum (Lonza), L-glutamine (2 mM), insulin (10 μg ml −1 ; I9278, Sigma) and 1% penicillin/streptomycin. SKOV-3 cells (ATCC) and U2OS cells (ATCC) were maintained in DMEM supplemented with 10% foetal bovine serum and 1% penicillin/streptomycin. To generate stable mESC lines, cells were transfected (TransIT-LT1; Mirus Bio LCC) with respective vectors and subjected to selection using G418 (Sigma, 300 μg μl −1 ) or puromycin (Sigma, 3 μg ml −1 ). Oct4 pseudogenes analysis and sequencing Genome blast analysis ( http://blast.ncbi.nlm.nih.gov/ ) was performed to identify mouse genomic regions with high similarity to Oct4 ( mus musculus Pou5f1 , transcript variant 1; NM_013633.3) mRNA. Genomic coordinates of identified pseudogenes were obtained using the University of California Santa Cruz (UCSC) genome browser. All candidate pseudogenes were PCR amplified from mESC cDNA using specific primers ( Supplementary table 1 ). PCR amplicons were cloned into pCR2.1-TOPO vector (Life Technologies) and subjected to bi-directional sequencing. Oct4P4-MS2 tethering model system To generate the Oct4P4-24 × MS2 stem loop construct, 24 repeats of the MS2 stem loop RNA motif (obtained from pSL-MS2-24 × , ref. 61 ) were cloned downstream of the Oct4P4 cDNA into pLPC. Oct4P4 cDNA was PCR amplified using the following oligonucleotides: forward: 5′-GGGAATTCAAGCTTGTCCCTAGGTGACCAACTCCT3′-; reverse: 5′-GGGAATTCAGATCTTGTGTCCCAGGCTTTTTAAA3′-). pCMV-FLAG-MS2nls was provided by A. Marcello (ICGEB, Trieste, Italy). RNA immunoprecipitation Cells were cross-linked in culture medium with 1% formaldehyde for 10 min. After addition of 125 mM glycine (PBS), cells were washed twice in ice cold PBS. Cross-linked cells were scraped in RIPA buffer (50 mM Tris-Cl, pH 7.5, 1% Nonidet P-40 (NP-40), 0.5% sodium deoxycholate, 0.05% SDS, 1 mM EDTA,150 mM NaCl) and supplemented with protease inhibitors (Complete, Roche) and RNaseOUT (Invitrogen). After incubation at 4 °C for 20 min, the cell lysate was sonicated and centrifuged. The supernatant was pre-cleared for 1 h at 4 °C with protein A/G PLUS-Agarose (sc-2003; Santa Cruz Biotechnology), supplemented with yeast transfer RNA (0.1 mg ml −1 , Invitrogen) and incubated overnight at 4 °C with the following antibodies: mouse monoclonal anti-FLAG M2, clone M2 (2.5 μg ml −1 ; F1804; Sigma); mouse monoclonal anti-KMT1A/SUV39H1 (2.5 μg ml −1 ; ab12405; Abcam); mouse monoclonal anti-HA, (2.5 μg ml −1 ; clone HA-7, H9658; Sigma). RNA–protein complexes were recovered with protein A/G PLUS-Agarose beads and were washed six times in high-stringency RIPA buffer (50 mM Tris-Cl, pH 7.5, 1% sodium deoxycholate, 0.1% SDS, 1 mM EDTA, 1 M NaCl, 1 M urea and 0.2 mM phenylmethylsulfonyl fluoride). An aliquot of beads containing immunoprecipitatated samples were saved for western blot analysis. Remaining beads were resuspended in 50 mM Tris-Cl, pH 7.0, 5 mM EDTA, 10 mM DTT and 1% SDS and incubated at 70 °C for 45 min to reverse cross-linking. The immunoprecipitated RNA and the total RNA were extracted with the Qiazol lysis reagent (Qiagen), subjected to DNase treatment (Qiagen) and subjected to reverse transcription (Quantitect reverse transcription kit; Qiagen). The obtained cDNA used for quantitative real-time PCR (SYBR Green Universal PCR Master Mix, Applied Biosystems) on a StepOnePlus real-time PCR machine (Applied Biosystems). The oligos used for quantitative RT–PCR are reported below: Oct4P4: forward: 5′-TGGCACCTGGCTTTAGACTTT-3′; reverse: 5′-CCAGGCCAACTTAGGGCATT-3′. 24 × MS2-Oct4P4: forward: 5′-CACCACGGCTTTGGAGTTAAG-3′; reverse: 5′-CATTAGATCTTGTGTCCCAG-3′. Analysis of immunocomplexes by western blotting: input and immunocomplexes proteins were resuspended in SDS–PAGE sample buffer, boiled for 15 min and analysed by western blotting. Primary antibodies: mouse monoclonal anti-FLAG (1:1,000; clone M2, F1804); mouse monoclonal anti-KMT1A/SUV39H1 (1:500; ab12405); mouse monoclonal anti-HA, clone (1:1,000; HA-7, H9658) rabbit polyclonal anti-Oct4 (1:1,000; ab19857; Abcam); anti-actin (1:1,000; A2066; Sigma). Secondary antibodies coupled to horseradish peroxidase (1:1,000; A-6154; A-4416; Sigma) were used for signal detection. Chromatin immunoprecipitation Cells were cross-linked in culture medium with 1% formaldehyde for 10 min, neutralized using 125 mM glycine in PBS and washed in PBS. Nuclei were obtained by lysing scraped cells in hypotonic buffer (5 mM Pipes pH 6.8, 85 mM KCl, 0.5% NP-40 and protease inhibitors), followed by centrifugation. Nuclei were resuspended in RIPA 100 mM buffer (20 mM Tris-HCl pH 7.5, 100 mM NaCl, 1 mM EDTA, 0.5% NP-40, 0.5% Na-Deoxycholate, 0.1% SDS supplemented with protease inhibitors). Chromatin was sonicated to 500—800 bp average fragment size and pre-cleared for 1 h at 4 °C with protein A/G PLUS-Agarose (sc-2003). Agarose was removed by centrifugation and an aliquot of supernatant was taken as input. Chromatin was immunoprecipitated overnight at 4 °C with the following antibodies: mouse monoclonal anti-FLAG M2, clone M2 (2.5 μg ml −1 ; F1804); mouse monoclonal anti-KMT1A/SUV39H1 (44.1; 2.5 μg ml −1 ; ab12405); rabbit polyclonal anti-trimethyl-Histone H3 (Lys9) (2.5 μg ml −1 ; 07-442; Millipore); mouse monoclonal anti-HP1a, clone 15.19s2 (2.5 μg ml −1 ; 05-689; Millipore); rabbit polyclonal anti-trimethyl-Histone H4 (Lys20) (2.5 μg ml −1 ; 07-749; Millipore); rabbit polyclonal anti-trimethyl-Histone H3 (Lys27) (2.5 μg ml −1 ; 07-449; Millipore). As a negative control for immunoprecipitation, mouse monoclonal anti-HA, clone HA-7 (2.5 μg ml −1 ; H9658) was used. DNA–protein complexes were recovered with protein A/G PLUS-Agarose beads and washed with RIPA 100 mM buffer, RIPA 250 mM buffer (20 mM Tris-HCl pH 7.5, 250 mM NaCl, 1 mM EDTA, 0.5% NP-40, 0.5% Na-Deoxycholate and 0.1% SDS), LiCl solution (10 mM Tris-HCl pH 8.0, 1 mM EDTA, 250 mM LiCl, 0.5% NP-40 and 0.5% Na-Deoxycholate) and 1 × TE. RNase treatment was performed in 1 × Tris-EDTA (TE) for 30 min at 37 °C. Cross-linking was reversed by overnight incubation at 68 °C after adding an equal volume of proteinase K solution (200 mM NaCl, 1% SDS and 0.3 mg ml −1 proteinase K). Samples were resuspended in ddH 2 O after phenol/chloroform extraction and ethanol precipitation. Co-immunoprecipitated DNA was analysed by RT–PCR on a StepOnePlus real-time PCR machine, using SYBR Green Universal PCR Master Mix. The oligos used for quantitative RT–PCR are reported below. Dkk: forward: 5′-GGGAACCAGGGAAAGAGGA-3′; reverse: 5′-GGGAAATAGGCACCCGATAA-3′. Oct4 (primer A): forward: 5′-TGCACCCCCTCCTCCTAATCC-3′; reverse: 5′-CCCTAAACAAGTACTCAACCC-3′. Oct4 (primer B): forward: 5′-GTTGGGGGGTGGTTAGTGTCT-3′; reverse: 5′-CCACTCCTCAGTTCTTGCTTA-3′. ChIP data of Oct4 promoter regions were normalized against input and the Oct4 unrelated DKK gene. Transient transfection mESCs and pMEFs were transfected with siRNAs (final concentration, 30 nM) using Lipofectamine RNAiMAX (Life Technologies) according to the manufacturer’s instructions. siRNA oligonucleotide: mouse Oct4 (Thermo Scientific Dharmacon; sense sequence: 5′-CGGAAGAGAAAGCGAACUAUU-3′), mouse Suv39h1 (Thermo Scientific Dharmacon; sense sequence: 5′-CCAAUUACCUGGUGCAGAA-3′) mouse Oct4P4 (Thermo Scientific Dharmacon; sense sequence: 5′-GAGCAUGAGUGGAGAGGAA-3′) and mouse Oct4P4#2 (Eurofins Genomics; sense sequence: 5′-GCCUCUCUUAAGCACUGUA-3′). siGENOME Non-Targeting siRNA#1 (D-001210-01-20, Thermo Scientific Dharmacon) and AllStars Negative Control siRNA (1027281; Qiagen; siControl#2) were used as a negative controls. Transient transfections of plasmids for pMEFs and U2OS were performed using Lipofectamine 2000 (Life Technologies) according to the manufacturer’s instructions. Luciferase reporter assay The mouse Oct4 promoter, corresponding to 2.9 kb of genomic region upstream of the Oct4 ATG, was PCR amplified from mESC genomic DNA; forward 5′-GGGAATTCCTCGAGATTGTACGTAAGTACTTCAGA-3′; reverse, 5′-GGGAATTCAGATCTGGGGAAGGTGGGCACCCCGA-3′ oligonucleotides. For the mouse Oct4P4 promoter reporter construct, 1.8 kb fragment upstream the Oct4P4 gene was PCR amplified from mESC genomic DNA; forward: 5′-GGGAATTCCTCGAGCATATGTGTGTCAATCTTGTT-3′; reverse: 5′-GGGAATTCAGATCTGGGGAAGTTGGGCACCCCAAG-3′. Fragments were cloned into pGL3Basic (Promega) via XhoI and BglII restriction sites located upstream of the firefly luciferase gene and sequence verified. pcDNA3-HA-OCT4 is reported in ref. 22 . For luciferase reporter assays, 4 × 10 4 NIH-3T3 cells were transiently co-transfected with 400 ng of pGL3 promoter luciferase reporters and 40 ng of CMV-Renilla to normalize for transfection efficiency; when indicated, 400 ng of pCDNA3-HA-Oct4 or pCDNA3-HA vector, and 400 ng of pCDNA3-Oct4P4 or pCDNA3 vector were co-transfected. Transient transfections were performed using Lipofectamine 2000 according to manufacturer’s instructions. For luciferase reporter assays involving siRNAs, plasmid DNA was transfected first followed by siRNA transfection after a 16-h recovery period. Firefly/renilla luciferase activity was assayed 72 h after transfection using the Dual Luciferase Assay kit (Promega). Statistical analysis Each finding was confirmed by three independent biological replicates, unless specified. Error bars represent s.d. All P values were determined using two-tailed t -tests and statistical significance was set at P <0.05. The variance was similar between groups that we compared. Uncropped scans of the most important blots are shown in Supplementary Fig. 9 in the Supplementary Information section. How to cite this article : Scarola, M. et al. Epigenetic silencing of Oct4 by a complex containing SUV39H1 and Oct4 pseudogene lncRNA Nat. Commun. 6:7631 doi: 10.1038/ncomms8631 (2015).